Water tribology on graphene Classical experiments show that the force required to slide liquid drops on surfaces increases with the resting time of the drop, t rest , and reaches a plateau typically after several minutes. Here we use the centrifugal adhesion balance to show that the lateral force required to slide a water drop on a graphene surface is practically invariant with t rest . In addition, the drop’s three-phase contact line adopts a peculiar micrometric serrated form. These observations agree well with current theories that relate the time effect to deformation and molecular re-orientation of the substrate surface. Such molecular re-orientation is non-existent on graphene, which is chemically homogenous. Hence, graphene appears to provide a unique tribological surface test bed for a variety of liquid drop-surface interactions. We learn in basic physics courses that the frictional force is proportional to the load (the Amonton law [1] ). Tribology teaches us that the frictional force is proportional to the contact area, whereas the Amonton law is a special case for very rough surfaces in which the load is roughly proportional to the contact area [2] . Recently, it was shown that for drops on surfaces, the frictional force can be inversely proportional to the load if, for example, we compare sessile and pendant drops [3] , [4] . This peculiar behaviour is a result of enhanced intermolecular interactions at the three-phase contact line which dominates the frictional force for this system [3] , [4] . The Shanahan-de Gennes surface deformation at the three-phase contact line [5] , [6] re-orients the molecules resulting in a new distribution of functional groups between those on the surface and those buried deeper in the surface. This enhances the solid–liquid interaction and, hence, the drop’s friction or lateral force [3] , [4] . A requirement for this behaviour is that the solid surface be chemically heterogeneous so as to allow different distributions of chemical functional groups between those that are on the surface and those buried deeper in it. This effect is associated with a variety of phenomena including the marked differences between chemisorbed and physisorbed monolayers [7] and wetting transitions [8] with implications ranging from plant growth [9] through electrovariable optical components [10] to nanofiber membranes [11] , which are chemically heterogeneous. Graphene, however, manifests a chemically homogeneous solid surface with peculiar mechanical friction and wear properties [12] , [13] , [14] , [15] , [16] . In this paper, we show that for water drops on graphene, the retention force for sessile and pendant drops is equal within the experimental scatter. In addition, for most systems, the re-orientation process described above reaches a plateau typically after about 10–20 minutes [17] . Here we show that for graphene, there is no variation in the retention force for drop sliding as a function of the time the drop rests on the surface suggesting an instantaneous re-orientation process for graphene surfaces. We conclude that the homogeneous and stable nature of graphene excludes the possibility of time changes in the intermolecular interactions between the liquid and the solid surface. Therefore, the only position for the three-phase contact line to pin on the surface is at the boundaries where graphene domains that nucleated at two adjacent nucleation sites meet. These boundaries form a complex micrometric tessellation whose shape is irrespective of the contact line, and hence should reduce its smooth nature. Indeed, we see that for graphene, the three-phase contact line forms a serrated micrometric structure, which differs from the smooth line on other surfaces. Critical angular velocity for drop motion A novel way of studying liquid–solid interactions is possible by measuring the combination of centrifugal and gravitational forces that drive liquid drops on solid surfaces using the recently established centrifugal adhesion balance (CAB) [4] . With this device, it is possible to independently measure and manipulate normal ( f ┴ ) and lateral ( f || ) body forces acting upon the liquid drop. A schematic illustration of the CAB is shown in Fig. 1a . The setup consists of a centrifugal arm on which a closed chamber is attached. The arm rotates horizontally using a computer-controlled dc motor. On one side of the arm is a counterbalance. On the other side is the chamber plate, which can be fixed at any desired angle with respect to the axis of rotation. In addition, a charge-coupled device camera inside the CAB chamber records video signals of the system in real time [4] . 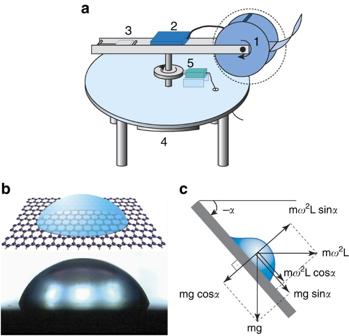Figure 1: Schematic illustration of the centrifugal adhesion balance and a water drop on graphene. (a) The CAB consists of a centrifugal arm with a closed chamber (1) at one end, a control box (2) in the middle and a counterbalance (3) on the other end. A drop is placed between a light source and a camera, all of which are housed in (1). The control box (2) obtains a signal from the camera and relays it wirelessly to a computer (not shown) located outside the pivoting assembly. The assembly is rotated using a dc motor (4). A round enlargement in the shaft is pressed against the encoder (5), which reads the angular velocity of the motor (4). (b) Top: schematics of a drop on graphene; bottom: a picture of a 10-μl water drop on graphene. (c) A vectorial representation of the forces acting on a drop in a tilted configuration of the CAB chamber (see equations 1 and 2). Note that α has a negative sign. Figure 1b shows a picture of a 10-μl water drop on a graphene surface (see characterization in Supplementary Fig. S1 (Raman spectra) and S2 (transmission electron microscopy (TEM))). 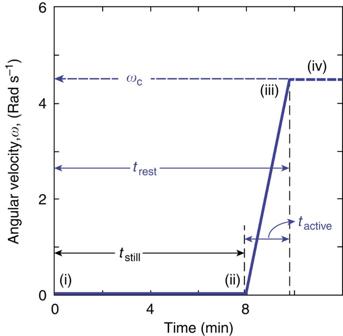Figure 2: Experimental procedure of a single-force datum measurement. The angular velocity acquired by the CAB,ω, is plotted against experimental time from the moment (t=0) the drop (V=6.5 μl) is placed on the graphene surface (G/2D=0.64).tstillis the period of time during which the CAB remains perfectly still (i)–(ii) withω=0.tactiveis the time at which theωis increased untilω=ωc, the critical angular velocity at which the drop begins to move (ii)–(iii). The total time the drop rests,trest, is the sum oftstillandtactive. This datum corresponds to the solid green circles inFig. 3b. Figure 2 shows how ω , the angular velocity of the CAB, is varied during a single measurement. Before rotating the CAB, different intervals of still time, t still , the time the drop is resting undisturbed in the motionless CAB chamber, (time period (i)–(ii) in Fig. 2 ) are maintained. Following t still , ω is gradually increased up to a critical value, ω c ((ii)–(iii) in Fig. 2 ) at which the drop starts sliding along the surface. Before reaching ω c , the drop is pinned to the surface but is slowly deformed in shape as the angular acceleration is increased. The time the drop is placed on the surface is time ‘zero’ in Fig. 2 . The resting time, t rest , is the time from which the drop is placed on the surface to when ω c is reached. Figure 1: Schematic illustration of the centrifugal adhesion balance and a water drop on graphene. ( a ) The CAB consists of a centrifugal arm with a closed chamber (1) at one end, a control box (2) in the middle and a counterbalance (3) on the other end. A drop is placed between a light source and a camera, all of which are housed in (1). The control box (2) obtains a signal from the camera and relays it wirelessly to a computer (not shown) located outside the pivoting assembly. The assembly is rotated using a dc motor (4). A round enlargement in the shaft is pressed against the encoder (5), which reads the angular velocity of the motor (4). ( b ) Top: schematics of a drop on graphene; bottom: a picture of a 10-μl water drop on graphene. ( c ) A vectorial representation of the forces acting on a drop in a tilted configuration of the CAB chamber (see equations 1 and 2). Note that α has a negative sign. Full size image Figure 2: Experimental procedure of a single-force datum measurement. The angular velocity acquired by the CAB, ω , is plotted against experimental time from the moment ( t =0) the drop ( V =6.5 μl) is placed on the graphene surface (G/2D=0.64). t still is the period of time during which the CAB remains perfectly still (i)–(ii) with ω =0. t active is the time at which the ω is increased until ω = ω c , the critical angular velocity at which the drop begins to move (ii)–(iii). The total time the drop rests, t rest , is the sum of t still and t active . This datum corresponds to the solid green circles in Fig. 3b . Full size image Retention force for graphene The normal and the lateral retention forces at ω c , (when the drop starts moving) are calculated (see Fig. 1c ) as follows: where m is the mass of the drop, g the gravitational acceleration, L is the distance of the drop from the axis of rotation and α the angle at which the CAB chamber plate is tilted with respect to the arm axis. A 0° tilt corresponds to a true sessile (+1 g) configuration and a 180° tilt corresponds to a true pendant (−1 g) configuration. Recent studies [4] , [17] show that the lateral force required for sliding drops on surfaces increases with the resting time. A schematic representation of this time effect is plotted in Fig. 3a , showing f || versus resting time. The force increases with resting time, and after some period, t pl , which is usually about 10–20 min (a time which is typical for re-organization of solid surface molecules [18] , [19] , [20] ), it reaches a plateau, denoted by t rest = t pl as demonstrated in Fig. 3a . We refer to the f || value that corresponds to t rest ≥ t pl as f ||pl . The trend shown in Fig. 3a is valid for a variety of drop-solid systems studied so far [4] , [12] , [17] , [21] , [22] , [23] . 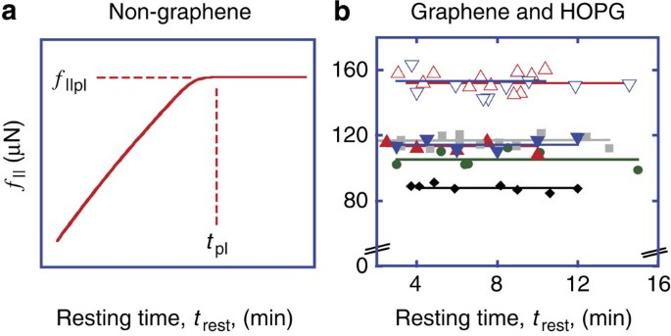Figure 3: Effect of time on drop retention force for various systems. (a) Schematic representation of the time effect showing a plot of lateral force,f||, required to slide a drop on a non-graphene surface, as a function of the drop-resting time,trest.f||plis the lateral force in the plateau region andtplis the time for the lateral force to reach the value off||pl. Usuallytpl~10–20 min for systems studied so far4,12,17,21,22,23. A few examples for such systems are shown inSupplementary Fig. S3. (b) Lateral force,f||, required to slide water drops on HOPG (solid grey squares) and graphene (other symbols) substrates as a function oftrest. Different symbols correspond to different substrate, drop volumesV, G/2D ratio and normal accelerations,a┴=(gcosα−ωc2Lsinα): solid black diamonds,V=4 μl, G/2D=0.64,a┴=−0.1±0.05g; solid green circles,V=6.5 μl, G/2D=0.64,a┴=0.22±0.04 g; hollow red triangle and hollow blue triangles,V=7 μl, G/2D=0.38, with hollow red triangles,a┴=−0.14±0.06 g, and hollow blue triangles,a┴=0±0.1 g; solid red triangles and solid blue triangles,V=7.5 μl, G/2D=0.83 with solid red triangles,a┴=+1 g (sessile) and solid blue triangles,a┴=−1 g (pendant); and solid grey squares,V=9.5 μl, HOPG substrate witha┴=+1 g (sessile). Figure 3: Effect of time on drop retention force for various systems. ( a ) Schematic representation of the time effect showing a plot of lateral force, f || , required to slide a drop on a non-graphene surface, as a function of the drop-resting time, t rest . f ||pl is the lateral force in the plateau region and t pl is the time for the lateral force to reach the value of f ||pl . Usually t pl ~10–20 min for systems studied so far [4] , [12] , [17] , [21] , [22] , [23] . A few examples for such systems are shown in Supplementary Fig. S3 . ( b ) Lateral force, f || , required to slide water drops on HOPG (solid grey squares) and graphene (other symbols) substrates as a function of t rest . Different symbols correspond to different substrate, drop volumes V , G/2D ratio and normal accelerations, a ┴ =( g cos α − ω c 2 L sin α ): solid black diamonds, V =4 μl, G/2D=0.64, a ┴ =−0.1±0.05g; solid green circles, V =6.5 μl, G/2D=0.64, a ┴ =0.22±0.04 g; hollow red triangle and hollow blue triangles, V =7 μl, G/2D=0.38, with hollow red triangles, a ┴ =−0.14±0.06 g, and hollow blue triangles, a ┴ =0±0.1 g; solid red triangles and solid blue triangles, V =7.5 μl, G/2D=0.83 with solid red triangles, a ┴ =+1 g (sessile) and solid blue triangles, a ┴ =−1 g (pendant); and solid grey squares, V =9.5 μl, HOPG substrate with a ┴ =+1 g (sessile). Full size image The effect of the resting time, t rest , on the lateral force, f || , required to set a water drop in motion on a graphene substrate is very different. Figure 3b shows that f || does not vary with t rest for water drops on graphene, regardless of the drop volume and the effective gravity the drop experiences, or the G/2D values characteristic of the graphene layer. Thus, f || ( t 1 )= f || ( t 2 )= f ||pl for graphene systems, where f || ( t 1 ) and f || ( t 2 ) represent f || values of any experimentally measurable resting times t 1 and t 2 . Similarly, highly oriented pyrolytic graphite (HOPG), whose surface has a similar chemical nature to that of graphene, exhibits the same behaviour. In addition to the time-independent behaviour of f || displayed in Fig. 3b , note that the f ||pl for sessile (+1 g) and pendant (−1 g) drops are similar for graphene surfaces (compare red up-triangles with blue down-triangles in Fig. 3b ) as opposed to the case of other known (and chemically heterogeneous), surfaces which exhibit significantly higher f ||pl for pendant drops [4] . The classic increase of f || as a function of the resting time shown in Fig. 3a has been theoretically related to the Shanahan-de Gennes deformation-induced re-orientation of the solid surface molecules [4] , [5] , [6] , [17] , which enables stronger intermolecular interactions of the re-oriented solid molecules with the liquid (hence, higher f || ). Such time dependence of f || is shown in Fig. 3a . For the graphene system shown in Fig. 3b , however, the general trend of Fig. 3a cannot be observed within the minimal time resolution of our experiments (to avoid drop motion due to pulsation, the change in ω 2 L needs to be gradual, leading to a minimal time of t active ~2 min to reach ω c sliding conditions). For an atomically homogeneous surface, such as the sp 2 carbon lattice in an ideal crystal of graphene (compare with Fig. 1b ), the molecular re-orientation can only be expressed in the realignment of the electronic orbitals, which is a phenomenon of the time order of attoseconds [12] . But if this was the mechanism associated with pinning the drop to the surface, then the slightest force aiming to slide the drop should have allowed the liquid molecules at the three-phase contact line to induce orbitalic re-orientation on the solid molecules nearby, and hence the sliding of the drop. In other words, there would be no force retaining the drop to the solid surface, although we know experimentally that this is not the case. Another mechanism to hold drops to a surface is via defects on the solid surface [24] . The liquid is either more energetically attracted to those defects compared with the rest of the surface or repelled by them. In either case, this creates a serrated three-phase contact line, which is then pinned to the defects either by adhering to them or by adhering to the rest of the surface and avoiding the defects. The defects on a graphene surface can emanate from the borders at the places where different domains of graphene that nucleated meet. Such junctions provide a morphologically different region and a ‘defect’ for the water drop to pin on. Studies carried out for understanding evolution and morphology of the chemical vapour deposition-grown graphene sheets revealed explicit domain structure [25] . Boundaries of the domains have mismatch in the atomic structure of the two meeting graphene layers, as well as Bernard stacking of the graphene layers as they overlap each other [26] . Further imperfections on the size scale of the droplet (ca. 10–100 μm) are also expected, for example, ripples [27] and point defects. The strength of the interaction with these defects has no time dependence, and hence we see straight horizontal lines in Fig. 3b . Although the regions of defects are difficult to resolve, such serrated three-phase contact line can be enhanced as the drop evaporates. 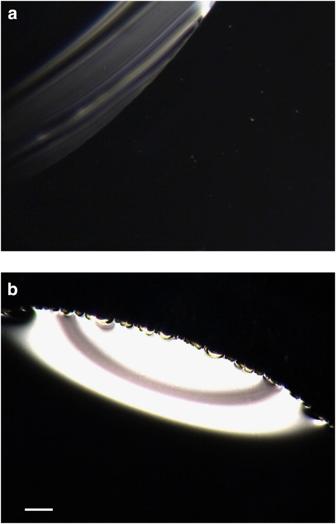Figure 4: Images of water drops on silane-treated silicon and graphene. Top view of a water drop on a (a) silane-treated silicon (b) graphene surface. The serrated three-phase line is evident on graphene, whereas on the non-graphene surface, the three-phase line appears smooth. The different light contrast corresponds to different light optimization for the different drop contact angles. Scale bar is 100 μm. Figure 4 shows that indeed the three-phase contact line of a graphene surface is serrated on a micron scale upon evaporation, whereas that of a non-graphene surface is not. Figure 4: Images of water drops on silane-treated silicon and graphene. Top view of a water drop on a ( a ) silane-treated silicon ( b ) graphene surface. The serrated three-phase line is evident on graphene, whereas on the non-graphene surface, the three-phase line appears smooth. The different light contrast corresponds to different light optimization for the different drop contact angles. Scale bar is 100 μm. Full size image The lack of time dependence in the drop-retention force shown in Fig. 3b is therefore a manifestation of the lack of any molecular re-orientation that can lead to a stronger solid–liquid intermolecular interaction of the liquid with the planar graphene surface. It should be noted that metals, being high-energy surfaces, have zero contact angle with almost any liquid [28] . In general, most hard surfaces are also high-energy surfaces because breaking the bonds of a hard material requires high energy. Graphene is an exception: on one hand it is hard and on the other hand, breaking the bonds between the layers, does not require as much energy. The deformation at the three-phase contact line that leads in other surfaces to molecular re-orientation of the solid molecules can only lead to topographic deformation in graphene, but not molecular re-orientation. The two energetically different states of graphene, the part inside the sheets and the part near their edges, have a chemical difference: the edges have dangling bonds, which are terminated by hydrogen atoms quickly after growth, whereas inside the sheets are composed of the classic sp 2 carbon lattice. All of these structures are already on the surface, and the mechanical strength and high-electrical conductivity of the graphene coating prevent any other functional groups located deeper in the substrate to re-orient, such as to reach the surface. Therefore, we see this peculiar tribological behaviour for graphene surfaces. The unique surface chemistry of graphene is also present in HOPG, and in Fig. 3b , we see that HOPG exhibits the same behaviour. This similarity supports attributing these tribological observations to the surface chemistry rather than deeper layers of the substrate. In addition to the previous observation on graphene substrates regarding the time dependency of f || , another interesting phenomenon observed in Fig. 3b is the similarity between f ||pl for sessile ( a ┴ =+1g) and pendant ( a ┴ =–1g) drops. In contrast, for non-graphene surfaces, the f ||pl for pendant drops is distinctively higher than that for sessile drops [4] . In the case of surfaces that consist of chemically heterogeneous molecules (that is, molecules with different chemical functional groups), the pinning force emanates from the enhanced intermolecular interaction associated with the deformation at the three-phase contact line. For pendant drops, higher f ||pl retention forces was attributed to gravity-induced facilitated three-phase contact-line deformation [3] , [4] , [23] . For the graphene sheet, however, the deformation of the surface does not affect its intermolecular interactions with the liquid. Therefore, the forces associated with sliding pendant and sessile drops are similar. In summary, using the CAB, we show experimentally that the retention force of water drops on graphene surfaces does not depend on the drop resting time, in contrast to any other known system. We further observe that the forces required to slide sessile and pendant drops on graphene sheets are similar. Both of these tribological observations are attributed to the chemical homogeneity and stability of graphene surfaces, which sustains the same morphology and chemical composition on the surface regardless of the Shanahan de-Gennes-type surface deformation. The retention force of the water drops on graphene surface is therefore only attributed to the boundaries where domains of graphene that nucleated at two adjacent nucleation sites meet. This gives rise to a unique serrated three-phase contact line on graphene surfaces. The three-phase contact line is pinned along the serrated structure of these domains and not to the Shanahan de-Gennes deformed ridge, and because the domains were on the surface historically, there is no time dependence to the drop-retention force on graphene. Materials Fabricated graphene based on the protocol of Srivastava et al [27] from Rice University was used. The distilled water used in the experiments was from Barnstead Nanopure Purification system, which provides specific conductance (at 25 °C) ≤0.7 × 10 −6 Ω −1 cm −1 . ParafilmM from Sigma-Aldrich was used as the goniometer sealing agent for all experiments performed using the CAB. HOPG grade SPI-1 (12 × 12 × 1 mm 3 ) was obtained from SPI Supplies and cleaved before use. We practiced slow cleaving of about 45 min for 1.4 cm 2 of HOPG surface. The silicon wafers (diameter: 76.2±0.3 mm; orientation: <110>±0.9°; resistivity: 0.0034–0.0046 Ω cm centre; thickness: 381±25 μm) used in this paper (obtained from Virginia Semiconductor) were cut into a 1.4 × 6-cm 2 piece, rinsed with ethanol, then with distilled water and dried in a StableTemp vacuum oven (model: 5053-10 from Cole-Parmer) at 100 °C for 30 min. Then it went through a 45 min cleaning using a ultraviolet/ozone Procleaner (model: Procleaner 110) to remove any organic impurities on the surface. From the ultraviolet/ozone cleaner, the silicon was immediately placed in a 1% (volume) solution of octadecyltrimethoxysilane (90% technical grade obtained from Sigma-Aldrich) in toluene (99.5% ACS Reagent obtained from Sigma-Aldrich), where it remained for 3 h at 70 °C. The surface was then washed with excessive amount of distilled water for at least 10 min, and was placed in a distilled water bath for about 45 min. Finally, it was dried in the vacuum oven at 80 °C for 15 min. Graphene preparation We fabricated graphene films using a protocol developed by Srivastava et al . [27] A 25-μm thick Cu foil substrate was loaded into quartz tube and the pressure was reduced to 10 −2 Torr before flowing in Ar/H 2 at a pressure of ~8–9 Torr. Heated to 950 °C in Ar/H 2 ambient and maintained for 30 min. The Ar/H 2 flow was stopped, and hexane vapour evaporated in situ from a liquid precursor (flow rate ~4 ml h −1 ) was passed in the quartz tube for 6 min. During the reaction time, we maintained tube pressure of 500 mTorr. Cu foils with the as-grown graphene films were spin-coated with a thin layer of poly methyl methacrylate (PMMA). Dilute nitric acid was used to dissolve the Cu foil. After dissolution, the PMMA-supported graphene was carefully washed with deionized (DI) water and transferred onto a silicon wafer capped with 300-nm silicon dioxide layer. The PMMA film was removed using acetone, leaving behind pure graphene on silicon wafer. To evaluate the number of graphene layers a Renishaw inVia spectrometer was used at 514.5 nm. Raman spectra of graphene are shown in Supplementary Fig. S1 . In addition, TEM image is shown in Supplementary Fig. S2 . Experimental procedure The CAB, used in this study, is described elsewhere [4] . Water drops were placed on the graphene substrate in a dust-free laminar flow hood (ULPA filters; Terra Universal) and then the drop-substrate system was carefully placed in the CAB chamber. To suppress the evaporation of the water, we placed several smaller (‘satellite’) water drops near the main (measured) drop and sealed the chamber as described previously [17] . Optical images of water drops on the graphene and silane-coated silicon were taken using Micromaster I microscope from Fisher Scientific. Raman spectroscopy Raman spectroscopy was used to measure graphene thickness and quality. A Renishaw inVia Microscope was set at 514 nm laser wavelength and at low 0.1 mW power to reduce sample heating. Graphene samples were mounted onto an n-type, 300 nm SiO 2 silicon wafer. For each sample, five different spots were measured and averaged into one curve. The intensity of disorder-induced Raman D-peak at ~1,350 cm −1 is weak, signifying high-quality graphene. The G (~1,595 cm −1 ) and 2D (~2,695 cm −1 ) are used to measure graphene layer number [29] ( n ) by comparing peak intensities, I ( G ) /I ( 2D ). TEM TEM was done using a JEOL 1,230 High Contrast Schottky-type field emission gun with a charge-coupled device Gatan model 794 camera. Power was at 120 eV and thermally induced drift was accounted for. Sample preparation was done by dispersing the graphene in 1:1 ethanol water mix and by placing a single drop on a 300-μm holey mesh lacey carbon grid with copper support. After drying, the grid was placed in the TEM chamber and measured. JEOL company software was used in image analysis. How to cite this article: N’guessan, H.E. et al . Water tribology on graphene. Nat. Commun. 3:1242 doi: 10.1038/ncomms2247 (2012).